Protein crystalline frameworks with controllable interpenetration directed by dual supramolecular interactions Protein crystalline frameworks are attractive for biomimetic and nanotechnological studies because they could augment the useful functionalities of numerous proteins through dense packing and uniform orientation. However, their formation and precise structural control is challenging. Here we present novel protein crystalline frameworks with controllable interpenetration. The homotetrameric lectin concanavalin A is crosslinked by predetermined inducing ligands containing monosaccharide and rhodamine groups connected by an oligo(ethylene oxide) spacer. Two non-covalent interactions, that is, sugar–lectin binding and the dimerization of RhB, are responsible for the framework formation. The three-dimensional structure of the framework is fully characterized by X-ray crystallographic methods. For the first time, either interpenetrating or non-interpenetrating frameworks are obtained, and they are controlled by the spacer length of the inducing ligand. Further kinetics and mechanistic investigations reveal that, in the self-assembly process, the carbohydrate–protein binding occurs first, followed by RhB dimerization. This sequence favours rapid crystallization with a high yield when an excess amount of inducing ligand is used. In short, by using well-controlled dual non-covalent interactions, fast and versatile preparation of protein crystalline framework was achieved with high crystallization ratio of the proteins, which may shed light on protein crystallization in near future. The self-assembly of proteins is a central and ubiquitous process in living systems and is responsible for the formation and development of varieties of one- (1D), two- (2D) and three-dimensional (3D) functional structures. Efficient examples are the large ribosomal heterocomplex, myosin filaments, crystalline bacterial S layers [1] and membranes containing 2D arrays of bacteriorhodopsin or porins [2] . In self-assembly studies with protein building blocks, various nanostructures, including vesicles and cages, fibres and tubes, and lattice patches on surfaces, have been reported [3] , [4] , [5] , [6] , [7] , [8] . However, discrete multidimensional architectures, that is, protein crystalline frameworks (PCFs) with regular lattice structures, are still rare compared with the large number of proteins. In fact, these frameworks are very special and attractive for biomimetic and nanotechnological studies as well as for further applications because they could augment the useful functionalities of numerous proteins through dense packing and uniform orientation [9] . X-ray diffraction has been a powerful tool for the study of PCF because it provides the most accurate details of the structure and the packing parameters of protein arrays [10] , [11] . However, the crystallographic research progress of PCF is, to some extent, restricted because very limited numbers of proteins naturally assemble to form crystalline frameworks and the process of formation of crystalline structures is typically extremely slow. Great effort has been devoted to the fabrication of protein crystals via, for example, fusing proteins to introduce required symmetry [2] , [7] , [8] or introducing small molecules to interact and link proteins [12] , [13] , [14] . An example of the outstanding progress achieved in recent years in this area is the strategy of metal-directed protein self-assembly, where protein–protein interaction is controlled through the introduction of metal coordination [10] , [15] . In this new strategy, surface modification of the proteins by genetic mutation, similar to that used for protein purification purposes, is necessary. PCFs strongly resemble metal–organic frameworks (MOFs), which are porous structures with a backbone of functional organic compounds connected with ligand–metal interactions, and have become a growing field in materials science [16] , [17] , [18] , [19] , [20] . In recent years, the interpenetration structure in MOFs, where two networks permeate each other, thereby reducing the porous density, has drawn great attention because it endows MOFs with certain valuable properties [21] , [22] . In fact, interpenetration is a basic structural feature of various materials, including minerals and even ice [23] , [24] . In addition, interpenetrating polymer networks have exhibited superior properties over their counterparts that are composed of simple blends, although they are usually in amorphous rather than crystalline states [25] . To our knowledge, interpenetrating structures in PCFs have not been reported. In this work, a novel approach to the fabrication of PCFs is presented where the key compound, referred to as the inducing ligand with monosaccharide and rhodamine groups connected by a oligo(ethylene glycol) spacer, is designed and employed. The inducing ligand connects the native protein concanavalin A (ConA) via dual supramolecular interactions, resulting in PCFs with and without interpenetration. This crystallization process includes features such as a rapid rate and high-yield production, which makes kinetic studies of the process and X-ray structure characterization of the resultant PCF proceed smoothly. Ligand structure and crystal generation To fabricate 3D protein frameworks with controllable interpenetration, lectin ConA, a homotetrameric protein exhibiting D2 symmetry, was selected. The tetramer contains four identical sugar-binding sites. To incorporate ConA into arrays, the inducing ligands shown in Fig. 1 were designed and prepared. The ligands contain three moieties: a sugar species of α- D -mannopyranoside (Man) or α- D -glucopyranoside (Glu), which is responsible for binding to ConA; rhodamine B (RhB), whose dimerization is due to π–π stacking connecting the ligand-attached ConA; and a short oligo(ethylene oxide) tether of varying lengths used to link the sugar and RhB. The inducing ligands are denoted as Rh n Man or Rh n Glu, where n is the number of ethylene oxide units. 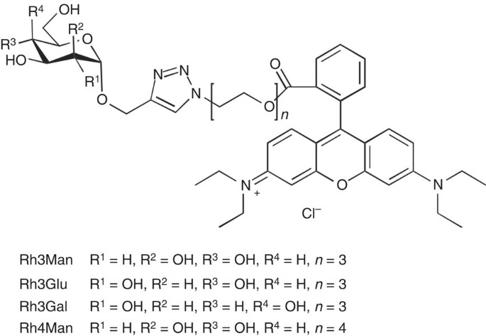Figure 1: Chemical structures of the inducing ligands. Rh3Man, Rh3Glu, Rh3Gal and Rh4Man. Figure 1: Chemical structures of the inducing ligands. Rh3Man, Rh3Glu, Rh3Gal and Rh4Man. Full size image The procedure to prepare protein crystals is simple: typically, equimolar quantities of Rh3Man were added to ConA in HEPES buffer ([HEPES]=20 mM, [NaCl]=100 mM, [CaCl 2 ]=5 mM, [MnCl 2 ]=5 mM); the final concentration of Rh3Man and ConA was 1.0 × 10 −4 M (ConA was calculated as a monomer in this work). The rapid generation of a large amount of pink crystalline material was subsequently induced. Crystallization then proceeded within a period of 30 min to several hours, depending on the salt concentration of the buffer. As shown in Fig. 2a–f , the resultant crystals exhibit relatively homogeneous squares with a side length of 10–100 μm. Lower NaCl concentrations and higher temperatures resulted in the formation of larger crystals. Atomic force microscopy observations of the crystal revealed a square geometry with flat surfaces and sharp edges ( Fig. 2g–j ). The height of the square was only ~200 nm. Control experiments designed by mixing ConA with different fragments of the inducing ligand—specifically, neat D -mannose, neat RhB, the spacer-attached α- D -mannose (EG 3 Man) and RhB (RhEG 3 N 3 ; Supplementary Fig. 1 )—did not exhibit any precipitation in any of the batches ( Fig. 1k ), indicating that the structure of Rh3Man in which RhB and Man moieties are connected is critical to this self-assembly process. Moreover, no precipitate was generated in the mixture of ConA and Rh3Gal ( Fig. 1 ), demonstrating that the specific interaction between Man and ConA is responsible for this self-assembly. 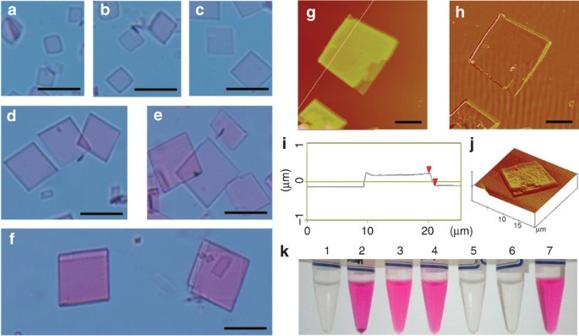Figure 2: Size control and characterization of the assemblies of ConA/Rh3Man complex. Different NaCl concentrations shown are (a) [NaCl]=100 mM, 5 °C; (b) [NaCl]=20 mM, 5 °C; (c) [NaCl]=0 mM, 5 °C; (d) [NaCl]=100 mM, 25 °C; (e) [NaCl]=20 mM, 25 °C; and (f) [NaCl]=0 mM, 25 °C. Atomic force microscopy height (g) and phase (h) images of the typical ConA/Rh3Man assembly with its cross-section profile (i) of the white line in the height image and (j) top view. (k) Control experiments for the assembly: 1.0 × 10−4M ConA (1) and those mixed with 1.0 × 10−4M of Rh3Man (2), RhB (3), RhEG3N3(4), EG3Man (5), Man (6) and Rh3Gal (7). Scale bar, 100 μm (a–f), 5 μm (g,h). Figure 2: Size control and characterization of the assemblies of ConA/Rh3Man complex. Different NaCl concentrations shown are ( a ) [NaCl]=100 mM, 5 °C; ( b ) [NaCl]=20 mM, 5 °C; ( c ) [NaCl]=0 mM, 5 °C; ( d ) [NaCl]=100 mM, 25 °C; ( e ) [NaCl]=20 mM, 25 °C; and ( f ) [NaCl]=0 mM, 25 °C. Atomic force microscopy height ( g ) and phase ( h ) images of the typical ConA/Rh3Man assembly with its cross-section profile ( i ) of the white line in the height image and ( j ) top view. ( k ) Control experiments for the assembly: 1.0 × 10 −4 M ConA (1) and those mixed with 1.0 × 10 −4 M of Rh3Man (2), RhB (3), RhEG 3 N 3 (4), EG 3 Man (5), Man (6) and Rh3Gal (7). Scale bar, 100 μm ( a – f ), 5 μm ( g , h ). Full size image Crystal structure of ConA/Rh3Man A large-size crystal was successfully obtained ( ca. 200 μm × 100 μm × 20 μm) and used for diffraction data collection, which was carried out at beamline BL14.1 of the BESSY II synchrotron facility [26] . The resulting structure provided clear evidence for the formation of a PCF. The structure, determined at 2.11 Å resolution ( Supplementary Table 1 ), consisted of Rh3Man molecules in a 1:1 molar ratio with ConA, which are present on each of the sugar-binding sites of the protein. The lattice parameter of the crystal was measured as a =84.00 Å, b =116.03 Å, c =84.10 Å, α =90.00°, β =95.03°, γ =90.00° with space group P 2 1 , as shown in Fig. 3a (the cell parameters are summarized in Table 1 ). As shown in Fig. 3 , intermolecular associations between ConA in the a – c plane are mediated entirely through the two different types of non-covalent interactions, that is, molecular recognition between ConA/Man and the dimerization of RhB ( Fig. 3c,d ), that is, the 2D lattice assembly of ConA in the a – c plane is only mediated by the connection of dimerized inducing ligand Rh3Man. Further information related to the crystal revealed that this connection is the only connection between neighbouring proteins in the a – c plane. The same lattice structures in different layers were then stacked along the b axis by limited protein contact close to the sugar-binding site. The junctions formed by the inducing ligands inside the crystal can be differentiated into two types, that is, ‘joint 1’ along the a axis (of ligand A′ on chain A and ligand B′ on chain B) and ‘joint 2’ along the c axis (of ligand C′ on chain C and ligand D′ on chain D); through joint 2, a given layer is attached to the other layer with protein contact. The configurations of inducing ligands are very similar between the two joint types ( Supplementary Fig. 2 ), except that only joint 2 is covered by ConA in the upper layer. In each binding site, the Man moiety fits into the pocket in the same manner as the ConA/α-mannopyranoside crystal [27] ; the subsequent triazole ring and the triethylene glycol spacer then form a helix-like structure. The triazole interacts with Tyr12 of ConA via a hydrogen bond between N5 and the phenol group (yellow dashed line in Fig. 3c,d ), which indicates that the configuration from Man to triazole is relatively rigid. The RhB group at the other end of the flexible triethylene glycol spacer forms a dimer with the RhB from the neighbouring inducing ligand. The stacking pattern of the RhB dimers differs from the H- and J-type dimers reported in the literature [28] , which could be the reason that the RhB dimer’s ultraviolet–vis absorption spectrum exhibited a similar, but not the same, peak shift, as discussed in detail in the Supplementary Information . In addition, the electron density analysis supports the interpretation that joint 1 is relatively broad compared with joint 2, indicating the relatively flexible nature of joint 1. 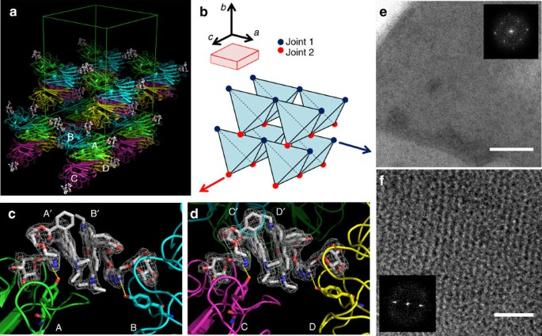Figure 3: Crystal structure of ConA/Rh3Man. (a) The packing of assembly of ConA/Rh3Man. The four monomers in a tetramer are represented with different colours; chain A (green), chain B (blue), chain C (purple) and chain D (yellow), and each tetramer is connected by Rh3Man dimers (shown in a stick model). The Rh3Man molecule binds to each of the four monomers of ConA, which are labelled as A′ (to chain A), B′ (to chain B), C′ (to chain C) and D′ (to chain D). The green cage represents the unit cell with a direction corresponding to the coordinate system shown inb. (b) The packing model of simplified tetrameric ConA with two different Rh3Man joints, specifically, joint 1 (blue corner) and joint 2 (red corner), with which ConA is crosslinked along the red and blue arrows, respectively. The selected layer represents the macroscopic form of the assembly, and the coordinate corresponds to that of the ConA packing models. Electron density (σ=1.5) and stick models of the Rh3Man at the Man-binding cites of (c) chain A/chain B and (d) chain C/chain D. The Tyr12 is shown as a stick model, which interacts with the triazole ring of Rh3Man as indicated by the yellow dashed line. (e) The molecular alignment in the assembly observed by transmission electron microscopy (TEM) by staining with uranyl acetate (scale bar, 500 nm); the 2D Fourier-transform image (2D-FFT) image is presented in the inset. (f) High-resolution TEM image of the isotopic protein alignment in the thin fragment of the assembly (scale bar, 50 nm); the 2D-FFT image is presented in the inset. Figure 3: Crystal structure of ConA/Rh3Man. ( a ) The packing of assembly of ConA/Rh3Man. The four monomers in a tetramer are represented with different colours; chain A (green), chain B (blue), chain C (purple) and chain D (yellow), and each tetramer is connected by Rh3Man dimers (shown in a stick model). The Rh3Man molecule binds to each of the four monomers of ConA, which are labelled as A′ (to chain A), B′ (to chain B), C′ (to chain C) and D′ (to chain D). The green cage represents the unit cell with a direction corresponding to the coordinate system shown in b . ( b ) The packing model of simplified tetrameric ConA with two different Rh3Man joints, specifically, joint 1 (blue corner) and joint 2 (red corner), with which ConA is crosslinked along the red and blue arrows, respectively. The selected layer represents the macroscopic form of the assembly, and the coordinate corresponds to that of the ConA packing models. Electron density ( σ =1.5) and stick models of the Rh3Man at the Man-binding cites of ( c ) chain A/chain B and ( d ) chain C/chain D. The Tyr12 is shown as a stick model, which interacts with the triazole ring of Rh3Man as indicated by the yellow dashed line. ( e ) The molecular alignment in the assembly observed by transmission electron microscopy (TEM) by staining with uranyl acetate (scale bar, 500 nm); the 2D Fourier-transform image (2D-FFT) image is presented in the inset. ( f ) High-resolution TEM image of the isotopic protein alignment in the thin fragment of the assembly (scale bar, 50 nm); the 2D-FFT image is presented in the inset. Full size image Table 1 Parameters determined by X-ray diffraction analysis of Rh3Man, Rh3Glu and Rh4Man. Full size table The feature of the unit cell in which assembled layers stack along the b axis provides a reasonable explanation for the formation of macroscopic thin squares. The transmission electron microscopy images in Fig. 3e show one corner of the crystalline square stained by uranyl acetate. Regularly aligned black dots were observed in two perpendicular directions, which was supported by the 2D Fourier-transform image. The aligned directions were parallel to the two sides of the square, and the distance between the dots was ~8 nm in both directions, corresponding to the cell parameter of the a and c axes (84.00 and 84.10 Å, respectively); hence, the b axis must be the normal direction of the square. Using a higher-resolution image analysis, we observed the dots to be aligned only in one direction, that is, the colour in one direction was much more intense than that in the other direction ( Fig. 3f ). Crystal structure of ConA/Rh3Glu To compare the effect of the binding ability of sugars on the formation of PCF, inducing ligand Rh3Glu was employed with the Glu moiety. This combination also resulted in crystalline protein arrays with a planar square shape ( Supplementary Fig. 3 ). Furthermore, the X-ray crystal structure showed that the crystal induced by Rh3Glu shares similar packing parameters with the crystal induced by Rh3Man ( Table 1 ), that is, the same space group ( P 2 1 ) with almost the same unit-cell parameters ( a =84.16 Å, b =116.01 Å, c =84.24 Å, α =90.00°, β =95.98°, γ =90.00°). In addition, the conformations of the Rh3Glu joints were almost the same as those of the Rh3Man joints because they share the same binding manner [29] , although the binding ability of the former is significantly weaker than that of the latter. The crystallization rate of ConA/Rh3Glu was, in fact, much slower than that of ConA/Rh3Man, which could be due to the weak interaction between ConA and Glu. Interpenetration in the crystal structure of ConA/Rh4Man Interpenetration of PCF was achieved when inducing ligand Rh4Man, in which the ethylene oxide spacer has four units, was employed. Using the aforementioned crystal formation procedure, we obtained PCF crystals induced by Rh4Man with a size and shape similar to that of the crystals induced by Rh3Man. However, the crystal formation of ConA/Rh4Man requires a substantially longer induction period, that is, several days, even at the highest salt concentration ([NaCl]=100 mM), and the number of obtained crystals was very limited. The X-ray analysis of the crystal structure of ConA/Rh4Man revealed that the structure crystallized in space group of P 2 1 2 1 2, with cell parameters of a =61.60 Å, b =116.11 Å, c =58.69 Å, α = β = γ =90.00°. Similar to the crystal induced by Rh3Man, the crystal structure induced by Rh4Man exhibited a 2D assembly in the a – c plane ( Fig. 4a ), with Rh4Man dimer joints ( Fig. 4c ) in the a and c axes. These layers were then stacked along the b direction ( Fig. 4b ). The most striking difference between the ConA/Rh4Man and the previous ConA/Rh3Man crystals is that the packing density of the ConA/Rh4Man is much higher; thus, its content of bulk water is only 39.1%, which is significantly smaller than the 68.7% bulk water content of ConA/Rh3Man. This greater packing density can be attributed to the number of ConA molecules per unit area of a single layer of ConA/Rh4Man being twice that of ConA/Rh3Man. As shown in Fig. 4b , in the crystal model of ConA/Rh4Man, two protein frameworks comprising blue-coloured ConA and red-coloured ConA coexist. The two frameworks are identical; however, they interpenetrate each other. Thus, different from the framework of Rh3Man, all of the Rh4Man dimers become joint 2 in the current framework. In addition, the absence of the crystal-twinning problem in ConA/Rh4Man (fraction=0.02 and 0.03, as shown in Table 1 ) was consistent with the fact that layer accumulation was supported by greater protein contact. 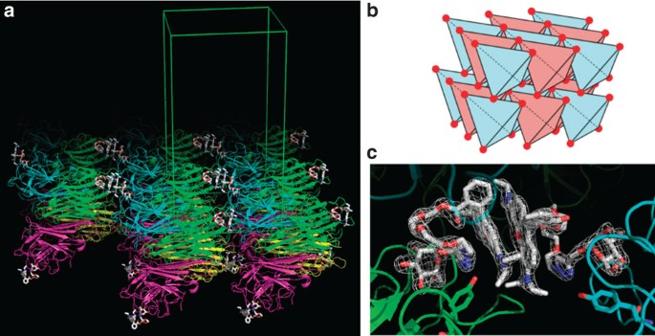Figure 4: The molecular packing of the ConA/Rh4Man crystal. (a) For clarity, only the molecules in one layer are shown. The layer stack in thebaxis direction in the real crystal. (b) The simplified packing model of ConA/Rh4Man. The red and blue colours of ConA are only for visualization; they indicate that the molecules of the same colour in a layer are crosslinked with each other via Rh4Man joints. (c) The conformation of the Rh4Man dimer joint. Figure 4: The molecular packing of the ConA/Rh4Man crystal. ( a ) For clarity, only the molecules in one layer are shown. The layer stack in the b axis direction in the real crystal. ( b ) The simplified packing model of ConA/Rh4Man. The red and blue colours of ConA are only for visualization; they indicate that the molecules of the same colour in a layer are crosslinked with each other via Rh4Man joints. ( c ) The conformation of the Rh4Man dimer joint. Full size image The molecular structures within one layer in the PCF of ConA/Rh3Man and ConA/Rh4Man are compared in Fig. 5 . Rh3Man induced a porous protein framework, whereas Rh4Man induced two interpenetrating frameworks, although each of the frameworks is very similar to that induced by Rh3Man. These results demonstrate that the presence or absence of an interpenetrating structure in PCF is controllable via a minor change in the structure of the inducing ligand. This change, of course, creates a new and interesting area of research for the construction of PCFs with desired structures and the exploration of their most suitable applications through changes in the structure of the inducing ligand. 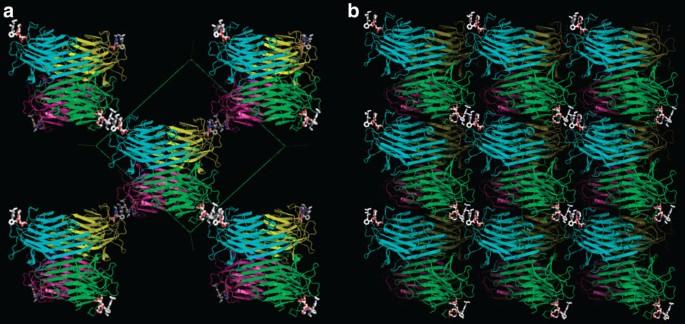Figure 5: The layer structures in the crystals viewed from the normal direction (baxis). (a) ConA/Rh3Man and (b) ConA/Rh4Man. Figure 5: The layer structures in the crystals viewed from the normal direction ( b axis). ( a ) ConA/Rh3Man and ( b ) ConA/Rh4Man. Full size image The unusually rapid protein crystallization for ConA with the inducing ligand enabled us to conduct a kinetic study, which served as a basis for understanding the crystallization mechanism. After mixing ConA (1.0 × 10 −4 M) with a threefold excess of Rh3Man (3.0 × 10 −4 M), the concentration profiles of both in solution were traced via ultraviolet–vis spectroscopy as a function of time. As shown in Fig. 6a , when almost all of the ConA precipitated within 1 h, the concentration of Rh3Man in the supernatant solution decreased by one-third and the rest of the ligand remained in the solution. Furthermore, as shown in Fig. 6b , the precipitation rate and amount (until the feeding concentration of ConA) increased monotonically with increased Rh3Man concentration, which allowed us to obtain a homogeneous assembly with a very rapid and high conversion rate just by adding an excess of Rh3Man to the protein solution. 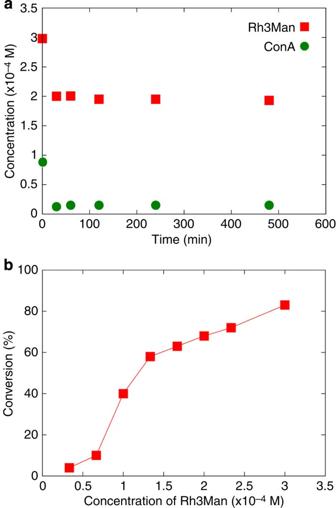Figure 6: Kinetic evaluation of ConA/Rh3Man crystallization. (a) The concentration profiles of ConA (square) and Rh3Man (diamond) as functions of time after the mixing of ConA (1.0 × 10−4M) and Rh3Man (3.0 × 10−4M). (b) Precipitated ConA versus the concentration ratio [Rh3Man]/[ConA]. Figure 6: Kinetic evaluation of ConA/Rh3Man crystallization. ( a ) The concentration profiles of ConA (square) and Rh3Man (diamond) as functions of time after the mixing of ConA (1.0 × 10 −4 M) and Rh3Man (3.0 × 10 −4 M). ( b ) Precipitated ConA versus the concentration ratio [Rh3Man]/[ConA]. Full size image On the basis of our study of the circular dichroism (CD) spectra ( Supplementary Fig. 4 ) and the fluorescence lifetimes ( Supplementary Fig. 5 ) of solutions of ConA and Rh3Man as functions of time, we concluded that, after being mixed with ConA, Rh3Man attaches immediately to the protein through Man/ConA binding and the dimerization of the RhB moiety subsequently occurs after an induction period, that is, the two supramolecular interactions occur in a cascade mode ( Fig. 7a ). This sequence enables the acceleration of the crystallization of ConA via the addition of an excess of inducing ligand, as shown in Fig. 6 . As shown in the scheme in Fig. 7a , the rapidly formed complex of the inducing ligand and ConA when the ligand is in excess would be connected by the subsequent dimerization. Conceivably, if the dimerization occurred before the binding, the binding sites of ConA would be occupied by the divalent ligand first, which would not have been able to be connected further ( Fig. 7b ). In the literature, divalent sugars have been reported to crosslink different lectin molecules to form crystals [12] . This behaviour is similar to the case described in Fig. 7b , where the efficiency of precipitation is limited because the molar ratio of protein and sugar should be exactly 1:1. The addition of an excess of linkers would further interfere with the crosslinking of the proteins because all of the binding sites have already been occupied. 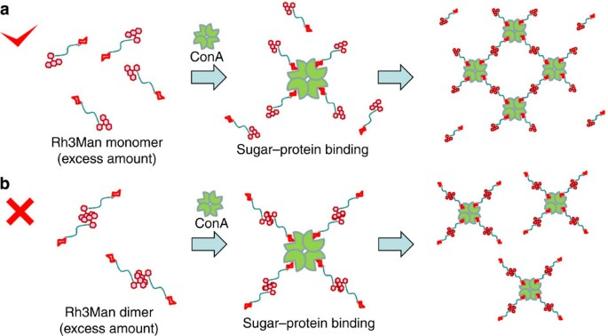Figure 7: Scheme of two possible sequences of Man/ConA interaction and RhB dimerization. (a) Rh3Man attaches to ConA first, followed by RhB dimerization, which leads to crosslinking. (b) Rh3Man forms a dimer first and then attaches to ConA. Here, the binding sites of ConA are occupied by dimerized Rh3Man; therefore, the occurrence of subsequent crosslinking is difficult. Figure 7: Scheme of two possible sequences of Man/ConA interaction and RhB dimerization. ( a ) Rh3Man attaches to ConA first, followed by RhB dimerization, which leads to crosslinking. ( b ) Rh3Man forms a dimer first and then attaches to ConA. Here, the binding sites of ConA are occupied by dimerized Rh3Man; therefore, the occurrence of subsequent crosslinking is difficult. Full size image Because of the rapid crystallization, direct monitoring of the heat associated with the crystallization process by calorimetry becomes possible. The heat released during protein crystallization is generally considered to be very small, and the crystallization is believed to be entropy driven [30] , [31] . Indeed, the solubility of a pure ConA crystal in the presence of poly(ethylene glycol) as a precipitant exhibited an inverse relationship with temperature [32] , which indicates that the enthalpy of crystallization has a positive value. However, in the present case of crystallization with the inducing ligand, a significant negative heat of approximately −63±5 kJ mol −1 (per mole of Rh3Man) was observed ( Supplementary Fig. 6 ). The enthalpy of the binding of ConA and Man was determined to be approximately −22 kJ mol −1 in our previous research [33] , and the heat generated by RhB dimerization was reported to be approximately −90 kJ mol −1 (per mole of RhB dimer, then 45 kJ mol −1 for one mole of RhB monomer) in the literature [34] . Thus, in the present case, the sum of these exothermal events (−22+(−45)=−67 kJ mol −1 ) is in good agreement with the heat released during crystallization. The favourable enthalpy clearly plays an important role in the ConA-inducing ligand crystallization. Further comparisons of the heat release between ConA/Rh3Man and ConA/EG 3 Man is discussed in the Supplementary Information . We observed that, in the a and c plane of the crystal structure, the lattice protein assembly was only induced by Rh3Man. On the basis of the CONTACT program in the CCP4 suite [35] , we listed contacting atom pairs (<3.9 Å) between two domains joined by inducing ligands ( Supplementary Table 2 , ConA/Rh4Man in Supplementary Table 3 ); we observed almost no direct contact between ConA. Obvious interactions other than RhB dimerization include the hydrogen bond between Tyr100 in chain A (chain C) and the oxygen of the xanthene group of ligand B′ (ligand D′; Supplementary Fig. 7 ). Moreover, the interaction between the layers maintained by protein contact at joint 2 appears to be weak and even tends to be misaligned. On the basis of such peculiar thermodynamics and structures, we believe that dimerization of RhB of the inducing ligand plays a key role in the assembly process; indeed, this role is easily verified by the addition of excess β-cyclodextrin, which breaks this linkage and triggers the immediate dissociation of the crystal ( Supplementary Fig. 8 ). In summary, new PCFs were prepared using natural protein ConA and small-molecular inducing ligands composed of sugar and rhodamine species connected by oligo(ethylene oxide). Crystallographic analysis revealed that the framework formation was promoted by the inducing ligand via dual supramolecular interactions and that the protein–protein contact within the framework is limited. The frameworks were able to form an interpenetrating structure, which has not been previously reported for protein crystals, depending exclusively on the tether length of the inducing ligands. Interpenetration is a well-known common feature in multidimensional structures in natural and synthetic materials, which bestows unique properties on the materials. Therefore, in these new PCFs, the exploration of interesting structural features as well as the rapid and convenient crystallization process with a significant contribution from enthalpy certainly depends on the interdisciplinary efforts of protein crystallography, supramolecular chemistry and materials science. Sample preparation The synthesis of inducing ligands is described in the Supplementary Methods ( Supplementary Figs 9–27 ). The sample solutions were prepared with HEPES buffer containing 20 mM HEPES, 5 mM CaCl 2 , 5 mM MnCl 2 and a desired concentration of NaCl, which was typically 20 mM. We prepared the ConA/Rh3Man mixture by mixing the ConA solution and Rh3Man solution. The ConA solution was prepared by dissolving ConA (lyophilized powder) in buffer and was stored overnight at 4 °C. Rh3Man was first dissolved in MeOH at a concentration of 10 −2 M as a stock solution, and the desired amount of the stock solution was subsequently transferred into tubes to remove the solvent, followed by the addition of buffer. The solutions were filtered through a 0.45-μm membrane filter (Millipore) before being mixed. Microscopy Optical microscopy was conducted with an Olympus BX53 equipped with an Olympus DR73 digital camera. The specimen was prepared by dropping the sample solution onto a glass plate, followed by direct observation. Transmission electron microscopy was performed on a JEOL JEM-2100F transmission electron microscope operated at an accelerating voltage of 200 kV. The samples were prepared by dropping the solution containing precipitates onto a copper grid and blotting the excess solvent; the samples were subsequently stained with a 1 wt% ethanol solution of uranyl acetate. Atomic force microscopy was performed on a Nanoscope IV digital instrument equipped with a silicon cantilever and an E-type vertical engage piezoelectric scanner. We prepared the sample by dropping the solution containing precipitates onto freshly cleaved mica. Spectrometry Ultraviolet–vis absorption spectra of the supernatant solution and precipitate dispersion were measured using a Shimadzu UV-2550 spectrophotometer. The supernatant solution was centrifuged at 6,000 r.p.m. for 5 min before measurement to completely remove the aggregated material. CD spectra were recorded on a JASCO J-810 CD spectrophotometer. Fluorescence lifetime studies were performed at λ em =595 nm on an Edinburgh FLS 920 photocounting system with a hydrogen-filled pulse lamp as the excitation source ( λ ex =510 nm); the data were analysed by iterative convolution of the luminescence decay profile with the instrument response function using the software package provided by Edinburgh Instruments. Dimerization of RhB group was characterized by ultraviolet–vis spectra in Supplementary Fig. 28 . Isothermal titration calorimetry Isothermal titration calorimetry experiments were conducted using a MicroCal VP-ITC system at 5.00±0.01 °C. The concentrations were 12.7 × 10 −4 M (1.8 × 10 −4 M after mixing) for the injected Rh3Man solution and 1.17 M (1.0 × 10 −4 M after mixing) for the ConA solution in the cell. Crystallography Because crystals for X-ray diffraction measurements were obtained by the diffusion method, 1.2 × 10 −4 M of the ConA buffer solution, pure buffer solution and 3 × 10 −4 M of ligand solution were sequentially loaded into a glass tube (diameter 3 mm) to a height of 40 mm and were left standing at ~25 °C. The NaCl concentration in the buffer was 20 mM for Rh3Man and Rh3Glu and 100 mM for Rh4Man (both including 20 mM HEPES, 5 mM CaCl 2 and 5 mM MnCl 2 , pH=7.2). We removed the crystals formed in the middle of the tube by cutting the tube with a glass cutter. Crystals suitable for diffraction experiments were transferred to a solution of mother liquor containing 4 M trimethylamine oxide [36] as a cryoprotectant, and they were subsequently flash frozen in liquid nitrogen. X-ray diffraction data were collected at beamline BL14.1 of BESSY II [26] , Helmholtz Zentrum Berlin, Germany, with 13.5 keV at 100 K. The diffraction images were integrated using X-ray Detector Software [37] , and the structures were determined by molecular replacement using MOLREP [38] . Rigid-body, positional, thermal and Translation Libration Screw refinement were conducted using REFMAC [39] , along with manual rebuilding with COOT [40] . All of the figures of the resulting structures were drawn using PYMOL ( http://www.pymol.org ). The bulk water content was calculated with the MATTHEWS_COEF program (MATTHEWS_COEF: a programme written by Misha Isupov) [41] , and the protein contact was determined using the CONTACT program in the CCP4 suite [42] . Accession codes: Coordinates for ConA/Rh3Man, ConA/Rh3Glu and ConA/Rh4Man have been deposited in the RCSB Protein Data Bank under accession codes 4P9W , 4P9X and 4P9Y , respectively. How to cite this article: Sakai, F. et al. Protein crystalline frameworks with controllable interpenetration directed by dual supramolecular interactions. Nat. Commun. 5:4634 doi: 10.1038/ncomms5634 (2014).